Topological solitons as addressable phase bits in a driven laser Optical localized states are usually defined as self-localized bistable packets of light, which exist as independently controllable optical intensity pulses either in the longitudinal or transverse dimension of nonlinear optical systems. Here we demonstrate experimentally and analytically the existence of longitudinal localized states that exist fundamentally in the phase of laser light. These robust and versatile phase bits can be individually nucleated and canceled in an injection-locked semiconductor laser operated in a neuron-like excitable regime and submitted to delayed feedback. The demonstration of their control opens the way to their use as phase information units in next-generation coherent communication systems. We analyse our observations in terms of a generic model, which confirms the topological nature of the phase bits and discloses their formal but profound analogy with Sine–Gordon solitons. Dissipative solitons have been observed in many nonlinear optical devices, both in the dimension transverse to light propagation and along the propagation dimension. Numerous examples have been found in nonlinear optical resonators with coherent forcing (they often receive the name of spatial or temporal cavity solitons) [1] , [2] , [3] , [4] , [5] , [6] but also in laser systems [7] , [8] , [9] , [10] . In the latter case, the phase of the electric field is free to evolve in the course of time and a paradigmatic model is the cubic-quintic Ginzburg–Landau equation [7] , [11] , [12] , [13] . On the contrary, the presence of an external field leads to the formation of dissipative solitons whose phase is locked to this external forcing in the second case, whose paradigmatic and first model is the Lugiato–Lefever equation [14] . In spite of this important difference [15] , the dissipative solitons observed in all of these systems are in most cases explained by a double compensation of dispersion (or diffraction) by Kerr nonlinearity and losses and gain [11] , [12] , [15] , [16] . In this work, we report on the experimental observation of dissipative optical localized states, which are fundamentally phase objects. Contrary to well-known dissipative optical solitons (phase-locked or not), the localized states we generate and control cannot exist in either of the paradigmatic models and their existence does not result from the usual double balance, but from the phase space topology of the system that supports them. Nevertheless, since they are attractors of a nonlinear and dissipative system, they share with usual dissipative solitons their discrete and robust character. These structures consist of self-localized 2 π phase rotations embedded in a homogeneously locked background field and therefore draw their robustness from their topological nature. Besides their fundamental novelty, their nature of phase objects and the possibility to nucleate and annihilate these states individually confer them exceptional properties as phase bits (Φ-bits), counterparts of the usual dissipative solitons as intensity bits. Owing to this, these Φ-bits bring the plasticity and robustness of optical localized states to the realm of phase information processing in coherent optical communication networks [17] , [18] , [19] . Experiment Our experiment is based on a semiconductor laser with coherent optical injection in a regime called excitable [20] , [21] , with the addition of a delayed feedback loop. A system is said to be excitable when any perturbation, which is sufficient to overcome the excitability threshold , elicits an always identical response, whose details do not depend on the perturbation. Paradigmatic examples include neural or cardiac cells [22] , [23] . In this configuration and without feedback, the phase of the semiconductor laser is stably locked to the external forcing, except when responding to a sufficiently large external perturbation [24] , which triggers a relative 2 π phase rotation after which the system locks again to the external forcing. We use the delayed feedback as a spatial degree of freedom [25] , [26] , [27] , [28] in which multiple independently addressable Φ-bits can be stored indefinitely. The experimental arrangement is shown on Fig. 1 . It consists of a single transverse and longitudinal mode semiconductor laser (called ‘slave laser’) under the action of coherent external forcing and delayed optical feedback. In order to obtain the desired phase space topology, the slave laser is biased at very high pump value (six to eight times the standalone lasing threshold, emitted power ~500 μW) and the master laser is tuned such that the detuning between both lasers is close to 5 GHz. The power of the injection beam (2–3 μW depending on realizations) is set such that the slave laser is in a stable stationary state in which its phase is locked to the external forcing. The injection beam detuning and power, together with the bias current of the slave laser, are chosen such that the system is excitable [24] . This parameter regime allows to essentially confine the dynamics in phase space on a circle whose radius is set by the emitted power and which contains two fixed points, one stable and one unstable, representing two different values of the relative phase of the slave laser with respect to the forcing. 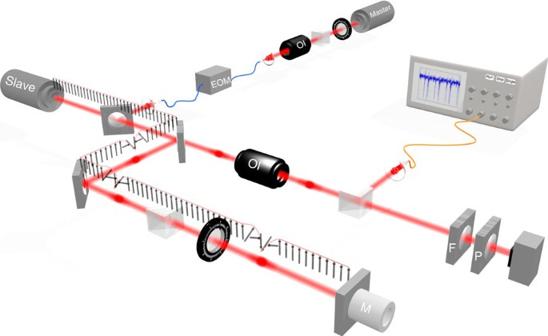Figure 1: Experimental set-up. The slave laser is submitted to optical injection by the master laser. Unidirectional coupling is ensured by an optical isolator (OI) and phase perturbations can be applied to the slave laser via the fibre-coupled electro-optic phase modulator (EOM). The arrows show a schematic view in theℜ(E),ℑ(E) plane of several Φ-bits stored in the feedback loop. Figure 1: Experimental set-up. The slave laser is submitted to optical injection by the master laser. Unidirectional coupling is ensured by an optical isolator (OI) and phase perturbations can be applied to the slave laser via the fibre-coupled electro-optic phase modulator (EOM). The arrows show a schematic view in the ℜ ( E ), ℑ ( E ) plane of several Φ-bits stored in the feedback loop. Full size image Perturbations can be applied to the system via a phase modulator. In order to confer the system an analogue of spatial degree of freedom, we place it inside an optical feedback loop. This is achieved by directing part of the emitted intensity towards a polarizer, quarter wave plate and high-reflectivity mirror that constitute a feedback loop of 0.5–1% reflectivity. The mirror is initially placed at a distance of ~30 cm and its subwavelength positioning is set via a piezoelectric actuator. The detection apparatus comprises a Fabry–Perot interferometer for spectral monitoring and a 9-GHz photodetector whose output is further amplified by a 14-GHz AC-coupled amplifier whose output is acquired via a 12.5-GHz bandwidth (100GS s −1 ) real-time oscilloscope. The detection is isolated from the experiment by a 30-dB optical isolator to prevent spurious reflections towards the slave laser. In absence of the optical feedback, the system responds to suitable phase perturbations [24] by emitting a single excitable pulse, which is a homoclinic orbit in phase space [20] . This pulse consists of the relative phase between slave and master laser completing a full circle before settling again to the initial value [24] , [29] , in excellent analogy with an overdamped pendulum submitted to a fluid torque [30] or excitable particles in an optical torque wrench [31] . Slow (>200 ps) or wrongly oriented phase variations do not trigger the excitable response [24] . This response is detected as a small pulse in the emitted power (10–25% of DC value depending on parameters). Experimental results In presence of very weak optical feedback with adequate phase, we observe that a pulse with essentially identical characteristics (amplitude and duration) is emitted, but also regenerated after a delay very close to the delay time. This observation is reported on Fig. 2a,b . 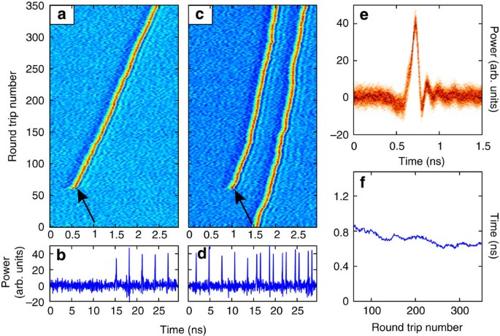Figure 2: Nucleation of two Φ-bits in space–time representation. (a) a phase perturbation is applied (black arrow) while the system is in a stable stationary locked state. Following that perturbation, a pulse is nucleated and repeats with a periodicity close to the feedback delay time, as shown inb. The space–time representation is chosen such that the pulse is almost stationary (see text). After some time a phase perturbation is applied again on the system (black arrow), with the first Φ-bit already stored. The two Φ-bits now propagate in the feedback loop, without perturbing each other (c,d). (e) superposition of a single Φ-bit waveform over 350 roundtrips. The very well-defined shape indicates the attractor nature of the Φ-bit. The ringing following the pulse is attributed to the detection set-up. (f) Evolution of the distance between the two pulses in the course of time. Figure 2b shows the time trace as measured by the detection apparatus; however, the trajectory of the pulse in the feedback cavity is best observed in the co-moving reference frame (see Methods), as shown in (a). On this graph, the horizontal axis is a space-like coordinate x (in nanoseconds) chosen such that the pulse is almost stationary and the vertical coordinate ξ (in units of x ) corresponds to the temporal evolution of the system over many round-trips. At this point, the possibility of using the spatial degree of freedom of the system to store information becomes clear. We show the first demonstration of this in Fig. 2c,d . The pulse created previously as shown in Fig. 2 is now at position x =1.5 ns at time ξ =0 and slowly drifting to the right. At round-trip number ξ =60 and space position about x =1 ns, a phase perturbation is applied on the injected beam via the phase modulator. As previously, this perturbation triggers a pulse, which is regenerated periodically due to the optical feedback. The mutual independence of these pulses demonstrates their nature of ‘localized structures’. Of the utmost importance, we underline that all the data shown in Fig. 2 consist of real-time data. This enables the measure of the speed of the pulses in the feedback loop (see Methods). Figure 2: Nucleation of two Φ-bits in space–time representation. ( a ) a phase perturbation is applied (black arrow) while the system is in a stable stationary locked state. Following that perturbation, a pulse is nucleated and repeats with a periodicity close to the feedback delay time, as shown in b . The space–time representation is chosen such that the pulse is almost stationary (see text). After some time a phase perturbation is applied again on the system (black arrow), with the first Φ-bit already stored. The two Φ-bits now propagate in the feedback loop, without perturbing each other ( c , d ). ( e ) superposition of a single Φ-bit waveform over 350 roundtrips. The very well-defined shape indicates the attractor nature of the Φ-bit. The ringing following the pulse is attributed to the detection set-up. ( f ) Evolution of the distance between the two pulses in the course of time. Full size image We analyse the evolution of the shape of a single Φ-bit in the course of time by plotting in Fig. 2e the superposition of a single Φ-bit over 350 round-trips. The very well-defined shape indicates the attractor nature of the Φ-bit. Finally, we show in Fig. 2f the evolution of the distance between the Φ-bits over successive round-trips. Again, the slow evolution of the distance is a confirmation of the interpretation of the Φ-bits in terms of mutually independent localized states and not simply a harmonic solution of the fundamental period set by the feedback loop. As becomes evident from Fig. 2 , independent topological localized structures can be juxtaposed only in a space which is large enough, otherwise interactions may set in. In the latter case all the peaks would move all together. This is illustrated in Fig. 3a . In this case, seven Φ-bits have been stored in the memory. At about round-trip 100, the central structure vanishes spontaneously because of electronic noise in the bias current control system, which also perturbs the other Φ-bits. At that point, we observe that upon cancellation of one of the structures, the other structures smoothly reorganize, the fourth one drifting to the left, later followed by the fifth one. We notice that this reorganization does not consist of an abrupt reconfiguration of the ensemble, but a rather a slow motion of each pulse confirming their weak interaction. The fluctuating distances indicate the degrees of freedom associated with the separations between pulses, which we analyse theoretically as the last part of our results. 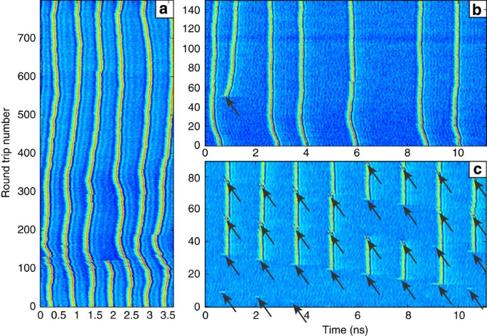Figure 3: Control of Φ-bits. (a) Seven Φ-bits initially co-exist in the feedback loop. The six remaining bits reorganize in the course of time after cancellation of the central one. (b) Six Φ-bits are present in the feedback loop. A perturbation (black arrow) is applied and nucleates a seventh Φ-bit. The two nearest neighbour repel each other until they reach sufficient time separation (790 ps) but the other existing Φ-bits are not affected. (c) Many perturbations (black arrows) are applied successively in time and nucleate several Φ-bits starting from the homogeneous state. Existing Φ-bits can be canceled if they are hit by a phase perturbation as shown at approximate coordinates (6;40) and (8;40). In this case, a nonmonotonous sequence of 13 different 8-bit integers has been stored. The same perturbation parameters are used for nucleation and cancellation. Note that the feedback loop is three times larger inb,cthan ina. Figure 3: Control of Φ-bits. ( a ) Seven Φ-bits initially co-exist in the feedback loop. The six remaining bits reorganize in the course of time after cancellation of the central one. ( b ) Six Φ-bits are present in the feedback loop. A perturbation (black arrow) is applied and nucleates a seventh Φ-bit. The two nearest neighbour repel each other until they reach sufficient time separation (790 ps) but the other existing Φ-bits are not affected. ( c ) Many perturbations (black arrows) are applied successively in time and nucleate several Φ-bits starting from the homogeneous state. Existing Φ-bits can be canceled if they are hit by a phase perturbation as shown at approximate coordinates (6;40) and (8;40). In this case, a nonmonotonous sequence of 13 different 8-bit integers has been stored. The same perturbation parameters are used for nucleation and cancellation. Note that the feedback loop is three times larger in b , c than in a . Full size image In order to minimize the interaction between structures, the feedback loop must be much larger than many times the typical interaction distance. The experimental set-up is therefore modified to increase the available space and the feedback mirror is set at a distance of ~1.65 m. We show in Fig. 3 the addressing of many Φ-bits and show that they can exist at different distances from each other. We start ( Fig. 3b ) with six Φ-bits previously nucleated and co-existing in the cavity. At round-trip 50, a perturbation is applied that nucleates a new bit. This new structure is nucleated with a temporal separation of 570 ps from another existing structure. Consequently, the new structure is repelled from the nearest neighbour in a way that is strongly reminiscent of the ultraweak force between temporal cavity solitons [32] , [33] but in the present case we can attribute this interaction to the refractory time following excitable pulses [34] . This interaction lasts ~50 round-trips. At this point, the structures have repelled to a temporal separation of ~790 ps after which no strong repulsion is observed and the distance is essentially randomly fluctuating. The absence of interaction between the pulse is clear on top of 3(b), in which the structures are separated by arbitrary distances. Finally, we demonstrate the nucleation and annihilation of structures in Fig. 3c . To this aim, we repetitively apply phase perturbations at a repetition rate of 31.3 MHz, which trigger excitable pulses in different points of the space–time diagram, starting from an empty cavity (bottom of (c)). Some perturbations (at coordinates ( x , ξ )=(3.5;5), (2;8), (0.8;10), (10.5;12)) are hardly visible and did not nucleate structures due to fluctuations blurring the excitability threshold [24] , [31] . On the contrary, seven successful nucleations then take place and equally spaced pulses separated by ~1.5 ns in the feedback loop are generated. The eighth perturbation then appears again on the right of the co-moving reference frame and nucleates an eighth Φ-bit. At this point, we have demonstrated the co-existence of nine different solutions holding from 0 to 8 Φ-bits. The ninth perturbation arrives very close to an existing structure but does not perturb it strongly. On the contrary, the following two perturbations reach the system close enough to existing Φ-bits to annihilate them. Subsequent phase kicks do not perfectly superimpose with existing structures and therefore only perturb them without destroying them. From round-trips 40–60, the system has been switched to another existing state in which only 6 Φ-bits are present in the cavity. This state differs from the other 6-Φ-bits state that exists around round-trip 28 by the configuration of the bits. This configuration can contain information. At round-trip 62 and 64 new structures are nucleated again in the space that was previously freed by the cancellation achieved close to round-trip 40. It is of course difficult to annihilate these temporal localized states since applying a perturbation to them requires accurately aiming in time. In this case, we have achieved it by perturbing in a repetitive way at a period that is not too far from a multiple of the round-trip time. The result shown in Fig. 3 constitutes the first demonstration of optical annihilation of temporal localized states, and also a demonstration of the switching between many states including from 0 to 8 Φ-bits in different configurations. Theoretical analysis The experimental observations can be interpreted within the generic framework of the injected Ginzburg–Landau equation extended to the influence of a delayed feedback. The equation governing the evolution of the optical field E reads. In equation (1), time has been scaled to the photon lifetime in the cavity times the excess pumping above threshold, while α and Δ= ω L − ω Y stand for the linewidth enhancement factor and the detuning between the solitary laser frequency ω L and the injected field ω Y , respectively. The optical feedback E τ =( t − τ ) with time delay τ has an amplitude and a phase denoted η and Ω , respectively. The field amplitudes E and Y have been rescaled to the one of the solitary laser and by definiteness. Although such a model may not represent the whole complexity of the system, it can be derived rigorously from standard laser equations close to the threshold [35] . It is also one of the simplest paradigm that is able to capture the physics of the problem and the important ingredients of the phase space geometry. Importantly, it allows us to connect with the experimental results by noting that the output of the VCSEL consists of a superposition of the emitted and reflected fields, which reads A = E − kY with k =(1− r 1 r 2 )[(1− r 1 )(1+ r 2 )] −1 ~1 with r 1,2 >0 the resonant reflectivities in amplitude of the top and bottom distributed Bragg Reflectors. The value of k is deduced by solving exactly the wave propagation within the linear empty regions of the VCSEL as in ref. 36 (see Supplementary Note 3 ). Our results are summarized in Fig. 4a,c,e,g in which we represent the (residual) temporal evolution of the intensity as well as the phase dynamics of the output field in good agreement with the experimental results. We present as well in Fig. 4b,d,f,h the stability of such periodic solutions. The stability information was obtained via a partial diagonalization of the Monodromy operator (see Methods). The monodromy Matrix describes the evolution of a perturbation after a full period. A solution is stable if all the eigenvalues of , the so-called Floquet multipliers, correspond to damped motion, that is, Max| μ |≤1. Owing to the infinite number of Floquet multipliers in a delayed differential equation, we represented in Fig. 4b,d,f,h a histogram of the multipliers N ( μ ) for the sake of clarity. In any time-invariant dynamical system, a periodic solution must present a Floquet multiplier equal to the unity. Often termed the trivial multiplier, it merely represents the translational temporal invariance and physically amounts to ‘shifting’ the solution without having to pay an ‘energetic’ cost. The details of the temporal waveform (for example, with several peaks over one period) are irrelevant. Such trivial multiplier is visible for the single Φ-bit solution. However, we demonstrate in Fig. 4d,f,h that the solutions with N Φ-bits are much more than a single multipeaked periodic solution: they present not one but N multipliers clustered around μ =1. This fact has a profound impact on the dynamics as it implies that the N Φ-bits solution possesses N neutral modes, which is actually what one would expect for independent Φ-bits. We analysed the eigenvectors associated with the various neutral multipliers and found that they correspond to relative translations of each of the Φ-bits, thereby confirming their independence. 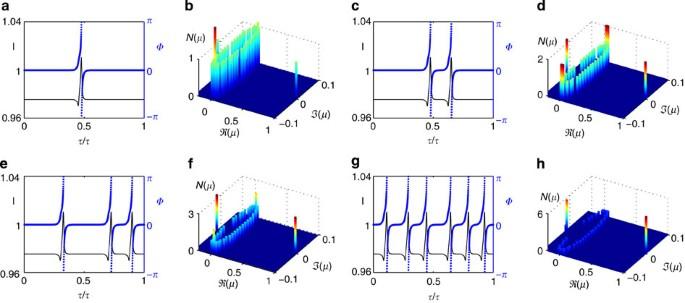Figure 4: Analysis of Ginzburg–Landau model with forcing and delayed feedback. Temporal traces (a,c,e,g) for the output intensityI=|A|2and phase Φ=arg(A) and histogramN(μ) of the Floquet multipliersμ(b,d,f,h) in the cases of 1, 2, 3 and 6 Φ-bits. One notices that the number of neutral modes located in the vicinity ofμ=1 increases linearly with the number of Φ-bits. The parameters areα=3, Δ=0.1,Y=2.9 × 10−2,η=5 × 10−3, Ω=0,k=1 andτ=2,000. Figure 4: Analysis of Ginzburg–Landau model with forcing and delayed feedback. Temporal traces ( a , c , e , g ) for the output intensity I =| A | 2 and phase Φ=arg( A ) and histogram N ( μ ) of the Floquet multipliers μ ( b , d , f , h ) in the cases of 1, 2, 3 and 6 Φ-bits. One notices that the number of neutral modes located in the vicinity of μ =1 increases linearly with the number of Φ-bits. The parameters are α =3, Δ=0.1, Y =2.9 × 10 −2 , η =5 × 10 −3 , Ω=0, k =1 and τ =2,000. Full size image For weak injection and detuning, one can, by applying a multiple timescale analysis to equation (1), reduce the problem even further to a single delayed equation for the phase (see Supplementary Note 1 ) that reads with θ =Φ+arctan α , , χ = η / Y and confirming that the dynamics consists essentially of a phase phenomenon. Interestingly, the same reduction to equation (2) is possible far from threshold from a full Class-B laser model with nonlinear gain compression in good correspondence with the experimental conditions. Such phase model allows us to exploit the strong link between delayed systems and spatiotemporal dynamics that was established in ref. 25 . By applying a multiple timescale analysis to equation (2) similar to the one in ref. 25 (see Supplementary Note 2 ), we formally reduce equation (2) to the modified Sine–Gordon equation with , x the pseudospace variable and ξ a slow temporal variable. When , analytical 2 π homoclinic orbits corresponding to kink solutions of this equation are known as In the general case, it was shown in ref. 20 that these homoclinic loops verify the Melnikov condition and therefore are robust in the limit and . They therefore persist in our case and we found that they seem to agree well with the numerical solutions of equation (2) even far from such perturbative limit. We demonstrated experimentally the optical control of independent phase bits in an excitable system with time-delayed feedback. We evidenced the nucleation of structures and analysed their basic interaction, which is repulsive, consistent with the underlying refractory tail of excitable pulses. The duration of each Φ-bit is close to 100 ps with typical interaction length less than 800 ps. Pulse of 70-ps duration (bandwidth-limited) was also observed. These values are basically set by the detuning between the slave laser and the external forcing. Since the Φ-bits are essentially phase objects, the semiconductor medium dynamics should not have a strong impact, and we expect that much shorter pulses could be realized with obvious benefits for information capacity. Finally, the nucleation of the Φ-bits was performed via phase perturbations; however, wavelength and intensity-phase conversions can be expected since excitable pulses in injection-locked semiconductor lasers can also be incoherently triggered [37] . The theoretical analysis, which has been presented, based on a generic model of a laser system with the addition of forcing and delayed feedback confirmed the paradigm that is required for the generation of Φ-bits, namely the presence of a saddle node on a circle bifurcation with the addition of a delay term. Owing to the simplicity of the model, we have been able to analyse numerically the neutral modes associated to the relative translation of the Φ-bits with respect to each other, which confirms their nature of localized states beyond the co-existence of multiple solutions, which was also observed. In addition, we exploited the strong relation between delayed and spatiotemporal systems, which allowed us to interpret the temporal Φ-bits as robust homoclinic kinks of a modified Sine–Gordon equation. Owing to the genericity of our results, we believe that next-generation photonic sources such as quantum cascade [38] or polariton [39] lasers may support Φ-bits with identical dynamical origin and features and very attractive physical properties. In conclusion, we have presented the first observation of temporal localized structures, which are topological in nature and thus essentially phase objects. These phase bits are attractors of an out-of-equilibrium system and they can be controlled independently of each other. As such, they can provide not only information storage, but also pulse reshaping and discrimination functionalities for the phase data which are the basis of coherent optical communication networks. Experimental set-up The laser used in the experiment is a Vertical Cavity Surface Emitting Laser (ULM980-03-TN-S46). It emits close to 980 nm in a single longitudinal and transverse mode and is linearly polarized up to 1.8 mA with coherent emission threshold at 0.2 mA. It is driven by a 1-μA resolution power supply and actively temperature-stabilized. The output of the Slave Laser is collected by a 4.5-mm focal length collimator. A half wave plate situated right after the collimator allows to align the polarization of the Slave Laser with the vertical axis. A 10% beam splitter is placed in front of it to serve as input for the Master Laser beam. The master laser is a tunable edge emitting laser with external grating in Littrow configuration. The amount of injected power can be precisely set via rotation of a half-wave plate placed between the master laser and a polarizer. The detuning between slave and master laser is set as Δ= ω L − ω Y >0. Phase perturbations can be applied to the system by applying voltage pulses to a fibre coupled 10-GHz lithium niobate phase modulator, which is driven by a 100-ps (10–90%) rise time pulse generator. The feedback cavity is not actively stabilized but is placed inside two layers of enclosure in order to avoid alterations of the feedback phase condition due to air circulation. Co-moving reference frame In order to clearly visualize the data, we process it such that the observer is in the co-moving reference frame of the Φ-bits. This is achieved by acquiring a single long enough time trace (in this case up to 10 7 points) and splitting this unique, perfectly synchronized time series into segments whose length corresponds to the time taken by a pulse to go to and back from the feedback mirror. The segments are then stacked on top of each other, so as to constitute a space-time diagram often used to analyse data in time-delayed dynamical systems [25] , [26] , [27] , [28] . In order for the pulses to be perfectly stationary, the length of the segments x must be x =τ+ δ where τ is the delay time. The additional delay δ results from the drift term of delayed dynamical systems [25] , [26] and from the fact that the Φ-bits, which are phase objects, may not propagate exactly at the group velocity, which is used to define τ . This procedure allows us to detect minute changes in δ that enables to observe, for instance, the synchronous change of direction of motion of all Φ-bits in Fig. 3b . Although we cannot separate the two terms contributing to δ , its total value in the parameter regimes used here has been found to be of the order of 12% of τ . On the other hand, τ was independently estimated by observing beat notes in nonstationary regimes and the modal structure of such aperiodic complex regimes could also slightly deviate from the exact time of flight in the external cavity. Numerical simulations The delayed differential equation given by the equation (1) was numerically integrated with a fourth-order Runge–Kutta method with constant step size ( δt =10 −2 ) (ref. 40 ). The delayed contribution in equation (1) demands a special care. To advance the solution with a step h from t n = nδt to t n +1 , the Runge–Kutta algorithm requires the values of E ( t − τ ) at intermediate points t n +1/2 . These are not known and must be interpolated from past values with an order of approximation consistent with that of the algorithm of integration. Therefore, besides keeping memory of the past values of E we also retain the past values of the time derivative . Such a method allows building a third-order Hermite polynomial approximation for E ( t ) between the time ( t n − τ ) and ( t n+ 1 − τ ). By evaluating this interpolating polynomial at ( t n+ 1/2 − τ ), we ensure an overall fourth-order accuracy. Stability analysis The linear stability analysis of the periodic solutions of equation (1) was performed via the reconstruction of the monodromy operator . Although a priori infinite dimensional, the operator reduces to a matrix of size τ / δt because of the discrete sampling incurred by the constant step-size numerical algorithm. Taking one point of the periodic orbit, we insert a small perturbation in all the degrees of freedom as represented by the mesh points in the delay time and let the system evolve over one period. The deviation of the end point from the unperturbed orbit yields a column of the operator . This method bears some similarity to the one developed in ref. 41 but here over a period and not a single time step. Owing to the large size , the eigenvalues and eigenvectors cannot be calculated from a complete decomposition using for instance the QR method [40] . Instead, we exploited the sparsity of and relied on the so-called Implicitly Restarted Arnoldi Method [42] searching for the eigenvalues of largest modulus. How to cite this article: Garbin, B. et al . Topological solitons as addressable phase bits in a driven laser. Nat. Commun. 6:5915 doi: 10.1038/ncomms6915 (2015).